HIV-1 Tat inhibits phagocytosis by preventing the recruitment of Cdc42 to the phagocytic cup Most macrophages remain uninfected in HIV-1-infected patients. Nevertheless, the phagocytic capacity of phagocytes from these patients is impaired, favouring the multiplication of opportunistic pathogens. The basis for this phagocytic defect is not known. HIV-1 Tat protein is efficiently secreted by infected cells. Secreted Tat can enter uninfected cells and reach their cytosol. Here we found that extracellular Tat, at the subnanomolar concentration present in the sera of HIV-1-infected patients, inhibits the phagocytosis of Mycobacterium avium or opsonized Toxoplasma gondii by human primary macrophages. This inhibition results from a defect in mannose- and Fcγ-receptor-mediated phagocytosis, respectively. Inhibition relies on the interaction of Tat with phosphatidylinositol (4,5)bisphosphate that interferes with the recruitment of Cdc42 to the phagocytic cup, thereby preventing Cdc42 activation and pseudopod elongation. Tat also inhibits FcγR-mediated phagocytosis in neutrophils and monocytes. This study provides a molecular basis for the phagocytic defects observed in uninfected phagocytes following HIV-1 infection. Macrophages are key components of the immune response. They are able to capture and degrade pathogens such as parasites or bacteria using several receptors that can be opsonic receptors such as those for the Fc of IgGs (FcγR) or for the complement protein iC3b (CR3), or pattern recognition receptors such as the mannose receptor (MR) [1] . Following the engagement of multiple receptors by the phagocytic target, the cell will initiate an intense and localized actin polymerization that is controlled by a distinct set of Rho GTPases, that is, Cdc42 and Rac1/2 for the FcγR, RhoA and RhoG for the CR3 (refs 1 , 2 ) and Cdc42 and RhoB for the MR-mediated phagocytosis [3] . This actin polymerization sustains the formation of membrane extensions called pseudopods that will engulf the target particle to form the phagosome. The phosphoinositide PI(4,5)P 2 seems to play multiple roles at the phagocytic cup, modulating actin polymerization by affecting actin-capping proteins [4] , regulating cytoskeleton plasma membrane adhesion [5] and enabling the recruitment of Rac1 and Cdc42 during FcγR receptor-mediated phagocytosis [6] . Although it can be strongly increased on opportunistic infection [7] , the proportion of infected macrophages in human immunodeficiency virus (HIV-1) infected patients usually ranges from 0.03 to 10% (refs 8 , 9 ). These low infection rates are consistent with the weak CD4 and CCR5 (that is, viral receptors) expression on macrophages [10] , and the presence in these cells of a resistance mechanism to HIV-1 infection based on the SAMHD1 protein [11] . Despite this partial resistance to infection and the low proportion of infected cells, phagocytosis is defective in macrophages from HIV-1-infected patients [8] , [9] , [12] . The other key phagocytes such as monocytes and neutrophils are, respectively, poorly (<1%) or not virally infected in HIV-1 patients. Nevertheless, their phagocytic activity is also affected in these patients [12] , [13] . Altogether these observations indicate that a secreted HIV-1 virulence factor might be responsible for the decreased phagocytic activity of phagocytes. This defect will allow the development of several opportunistic pathogens such as Toxoplasma gondii, Mycobacterium avium complex or Candida albicans. These infections are a major cause of morbidity and mortality during AIDS [8] , [9] , [12] . HIV-1 Tat strongly binds to PI(4,5)P 2 that enables its secretion directly through the plasma membrane of infected T cells [14] , generating Tat seric concentrations of 0.1–4 nM (refs 15 , 16 ). Circulating Tat is recognized by various cellular receptors that will enable it to enter uninfected cells by endocytosis before crossing the endosome membrane to reach the cytosol [17] . This transmembrane transport is triggered by endosomal low pH that induces Tat conformational modifications, allowing the exposure of Tat-single Trp (Trp11) that will initiate membrane insertion [18] . Tat translocation to the cytosol is catalysed by the molecular chaperone Hsp90 (ref. 19 ). Here we show that extracellular Tat at subnanomolar concentrations inhibits MR- and FcγR-mediated phagocytosis by entering macrophages and affecting the PI(4,5)P 2 -mediated recruitment and activation of Cdc42. Tat also inhibits FcγR-mediated phagocytosis in monocytes and neutrophils. Extracellular Tat is thus a secreted HIV-1 virulence factor that is able to interfere with the phagocytic activity of a wide range of phagocytes, thereby favouring the appearance and development of opportunistic infections. HIV-1 Tat inhibits phagocytosis in bystander macrophages Monocyte-derived human macrophages (MDMs) were infected with a macrophage-tropic virus (AD8) and cultured for 8 days before assaying FcγR phagocytosis using human-IgG-coated latex beads [20] . Infected macrophages phagocytosis efficiency was reduced by 50–60% ( Fig. 1a ). The Tat-W11Y mutant lacks the single Trp needed for Tat binding to PI(4,5)P 2 and for Tat transmembrane transports while maintaining a native Tat conformation. It is not secreted [17] . As observed before in T cells for the T-tropic virus [14] , the introduction of the Tat-W11Y mutation in the Ad8 M-tropic virus affected neither its ability to multiply in macrophages (4–8% of infection were reached during these experiments), nor the capacity of the virus to inhibit phagocytosis in infected cells. Tat-PI(4,5)P 2 interaction is, therefore, not involved in HIV-1-mediated phagocytosis inhibition in infected cells; we will come back to this point in the Discussion section. 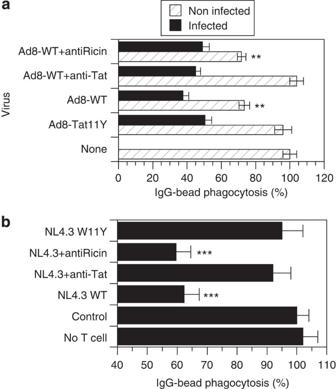Figure 1: HIV-1 Tat is responsible for phagocytosis inhibition in bystander macrophages. (a) Human primary macrophages (MDMs) were infected (multiplicity of infection (MOI) 0.5) with an M-tropic (Ad8) virus, bearing either WT Tat or Tat-W11Y. Antibodies (10 μg ml−1) were added to the medium as indicated. After 8 days (4–8% of infected cells), the phagocytosis of human-IgG-coated latex beads (3 μm diameter) was assayed. Extracellular beads were labelled on ice before cell fixation and infected cell detection using p24 antibodies. (b) CD4+T cells were purified, stimulated for 6 days then infected (MOI 0.5) with a T-tropic (NL4.3) virus, bearing either WT Tat or Tat-W11Y. After 1 day, T cells were washed then added to Transwells into wells containing autologuous MDMs (10 T-cells per MDMs). Cells were cocultured for 8 days before assaying FcγR-mediated phagocytosis. After this time, 20–35% of T cells and 0% of macrophages were infected. Data are mean±s.e.m. of three independent experiments (countingn>100 cells) and the significance of differences with control uninfected macrophages was assessed using an unpaired, two-sided Student’st-test (***P<0.001; **P<0.01). Figure 1: HIV-1 Tat is responsible for phagocytosis inhibition in bystander macrophages. ( a ) Human primary macrophages (MDMs) were infected (multiplicity of infection (MOI) 0.5) with an M-tropic (Ad8) virus, bearing either WT Tat or Tat-W11Y. Antibodies (10 μg ml −1 ) were added to the medium as indicated. After 8 days (4–8% of infected cells), the phagocytosis of human-IgG-coated latex beads (3 μm diameter) was assayed. Extracellular beads were labelled on ice before cell fixation and infected cell detection using p24 antibodies. ( b ) CD4 + T cells were purified, stimulated for 6 days then infected (MOI 0.5) with a T-tropic (NL4.3) virus, bearing either WT Tat or Tat-W11Y. After 1 day, T cells were washed then added to Transwells into wells containing autologuous MDMs (10 T-cells per MDMs). Cells were cocultured for 8 days before assaying FcγR-mediated phagocytosis. After this time, 20–35% of T cells and 0% of macrophages were infected. Data are mean±s.e.m. of three independent experiments (counting n >100 cells) and the significance of differences with control uninfected macrophages was assessed using an unpaired, two-sided Student’s t -test (*** P <0.001; ** P <0.01). Full size image Phagocytosis efficiency was also reduced by ~25% in uninfected macrophages from infected wells. This inhibition was not observed when a virus with a non-secreted Tat (Ad8-Tat-W11Y) was used or when anti-Tat antibodies were added to the medium, while it was still observed when irrelevant antibodies (that is, anti-ricin) were used. These results indicated that secreted Tat is responsible for phagocytosis inhibition in bystander macrophages. To confirm these findings, and since most HIV-1-infected cells are T cells [21] , we infected T cells with a T-tropic (NL4-3) virus, then added infected T cells to Transwells in plates containing autologous macrophages. After 8–9 days of coculture, FcγR phagocytosis was assayed. This coculture system enables to obtain stronger viral production and higher extracellular Tat levels. We did not detect macrophage infection under these conditions but phagocytosis was inhibited by ~40% when a native virus, but not when a virus with a non-secreted Tat (NL4-3-Tat-W11Y) was used ( Fig. 1b ). Addition of anti-Tat antibodies to the medium did not significantly affect viral production ( n =3 experiments) but prevented infected T cells from affecting phagocytosis by cocultivated macrophages. Control antibodies had no effect ( Fig. 1b ). Hence, secreted Tat is responsible for the inhibition of FcγR phagocytosis observed in these biologically relevant culture systems. We then used biologically active recombinant Tat [19] to study in more details Tat effect on phagocytosis. Tat strongly inhibits phagocytosis on cytosolic delivery The capacity of human MDMs to perform FcγR phagocytosis was inhibited up to 50% after macrophage treatment with recombinant Tat ( Fig. 2a ). This effect was already observed when using 0.2 nM Tat, a concentration within the low range of those found in the sera of HIV-1-infected patients (0.1–4 nM) (refs 15 , 16 ) and was maximum after only 2–3 h of contact ( Fig. 2b ). The Tat-W11Y mutant that cannot access the cytosol [18] did not affect phagocytosis, indicating that Tat cytosolic delivery is required to inhibit the FcγR-mediated phagocytosis. Similar dose–response and kinetics curves were obtained when we examined the effect of Tat on the phagocytosis of zymosan ( Fig. 2c,d ), which is essentially phagocytosed by the MR pathway in human macrophages [22] . We also assessed whether phagocytosis inhibition by Tat is reversible. Tat inhibitory effect on phagocytosis was still observed following cell washes, but was reversible following MDM culture for 2 days in the absence of Tat ( Supplementary Fig. 1 ). 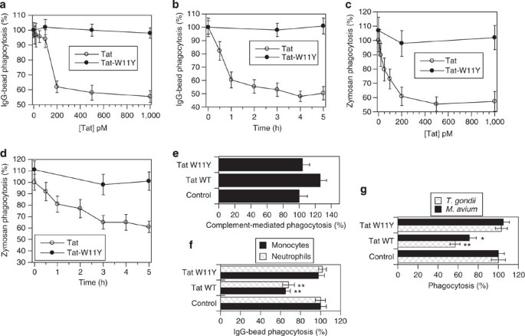Figure 2: Extracellular HIV-1 Tat inhibits FcγR- and MR-mediated phagocytosis on cytosolic delivery. (a) MDMs were treated with the indicated concentration of Tat WT or Tat-W11Y for 6 h at 37 °C before assaying IgG-bead phagocytosis. (b) Human MDMs were treated with 2 nM Tat or Tat-W11Y for the indicated time before IgG-bead phagocytosis assay. (c) MDMs were treated with Tat WT or Tat-W11Y for 6 h at 37 °C before assaying zymosan phagocytosis. (d) Human MDMs were treated with 2 nM Tat or Tat-W11Y for the indicated time before zymosan phagocytosis assay. (e) MDMs were treated with 10 nM Tat WT or Tat-W11Y for 6 h at 37 °C before pretreatment with PMA to assay complement-mediated phagocytosis using C3bi-coated beads. (f) Monocytes and neutrophils were purified from normal human blood and pretreated with with 2 nM Tat or Tat-W11Y for 5 h before assaying IgG-bead phagocytosis. (g) MDMs were treated with 2 nM Tat WT or Tat-W11Y for 6 h at 37 °C before assaying phagocytosis ofM. aviumor opsonizedT. gondii.Phagocytosis of unopsonizedT. gondiiwas negligible (~6% of opsonized control). Representative images are shown inSupplementary Fig. 3. Data are mean±s.e.m. of three independent experiments (countingn>100 cells) and the significance of differences with control cells was assessed using Student’st-test (**P<0.01; *P<0.05). Figure 2: Extracellular HIV-1 Tat inhibits FcγR- and MR-mediated phagocytosis on cytosolic delivery. ( a ) MDMs were treated with the indicated concentration of Tat WT or Tat-W11Y for 6 h at 37 °C before assaying IgG-bead phagocytosis. ( b ) Human MDMs were treated with 2 nM Tat or Tat-W11Y for the indicated time before IgG-bead phagocytosis assay. ( c ) MDMs were treated with Tat WT or Tat-W11Y for 6 h at 37 °C before assaying zymosan phagocytosis. ( d ) Human MDMs were treated with 2 nM Tat or Tat-W11Y for the indicated time before zymosan phagocytosis assay. ( e ) MDMs were treated with 10 nM Tat WT or Tat-W11Y for 6 h at 37 °C before pretreatment with PMA to assay complement-mediated phagocytosis using C3bi-coated beads. ( f ) Monocytes and neutrophils were purified from normal human blood and pretreated with with 2 nM Tat or Tat-W11Y for 5 h before assaying IgG-bead phagocytosis. ( g ) MDMs were treated with 2 nM Tat WT or Tat-W11Y for 6 h at 37 °C before assaying phagocytosis of M. avium or opsonized T. gondii. Phagocytosis of unopsonized T. gondii was negligible (~6% of opsonized control). Representative images are shown in Supplementary Fig. 3 . Data are mean±s.e.m. of three independent experiments (counting n >100 cells) and the significance of differences with control cells was assessed using Student’s t -test (** P <0.01; * P <0.05). Full size image Regarding CR3-mediated phagocytosis, we found that Tat, even at high concentration (10 nM) does not affect phagocytosis of complement-coated latex beads ( Fig. 2e ). Altogether, these results indicated that Tat specifically affects MR and FcγR-mediated phagocytosis. Tat does not affect the expression of phagocytic receptors Because Tat is known to inhibit transcription of the MR [23] , we examined whether Tat affected its ectopic expression in MDMs. We did not observe any significant effect ( Supplementary Fig. 2a ), indicating that Tat does not inhibit zymosan uptake through MR downregulation. Throughout this study we never observed that Tat significantly affected the binding of IgG-coated targets. To examine this point more directly, we tested the effect of Tat on the expression of the FcγRI receptor (CD64), a major phagocytic receptor in MDMs [24] . We did not find that Tat significantly modified the level of FcγRI in these cells ( Supplementary Fig. 2b ). Hence, Tat does not seem to perturb phagocytosis by affecting the ectopic expression of the MR and FcγRI phagocytic receptors. Tat inhibits FcγR phagocytosis in neutrophils and monocytes We then examined the effect of Tat on other key phagocytes, that is, monocytes and neutrophils. These cells do not significantly express the MR [25] . Tat inhibited FcγR-mediated phagocytosis in these cell types by ~40% ( Fig. 2f ), just as is the case for macrophages ( Fig. 2a,b ). Tat is thus able to affect phagocytosis in a wide range of different phagocytes. Tat inhibits phagocytosis of opportunistic pathogens To confirm these findings in a biologically relevant context, we used MDMs and pathogens that are a major cause of opportunistic infections in HIV-1-infected patients. M. avium complex infection is one of those and is a high risk for patients with low CD4 cell counts [26] . Phagocytosis of M. avium by rat alveolar macrophages was found to be inhibited by ~45% by mannan, indicating that uptake of this pathogen largely relies on the MR [27] . We accordingly observed using MDMs that mannan inhibited M. avium phagocytosis by 60–66% (mean±s.e.m. from n =3 experiments). Interestingly, it was previously observed that HIV-1 infection of MDMs decreased phagocytosis of M. avium by ~40% (ref. 28 ). In agreement with this observation, we found that Tat, but not Tat-W11Y, inhibited phagocytosis of M. avium by ~30% ( Fig. 2g and Supplementary Fig. 3 ). The incidence of cerebral toxoplasmosis in HIV-1-infected patients is also inversely correlated with CD4+ T-cell counts [29] and is most often due to reactivation of latent infection in patients seropositive for T. gondii [30] . It was earlier shown that HIV-1 infection of macrophages impairs T. gondii phagocytosis [31] . We first compared the efficiency of MDM invasion by unopsonized parasites with the efficacy of FcγR-mediated phagocytosis of opsonized T. gondii , and found that invasion was negligible (~6% of phagocytic uptake). We then examined the effect of Tat and observed that Tat inhibited phagocytosis of opsonized T. gondii by 40% ( Fig. 2g and Supplementary Fig. 3 ). Tat-W11Y did not have any effect. Hence, Tat is able to impair phagocytosis of opportunistic pathogens captured using the FcγR- (opsonized T. gondii ) or MR pathway ( M. avium ). Tat is delivered to the cytosol following endocytosis Data obtained using the W11Y mutant indicated that Tat had to reach the cytosol to inhibit phagocytosis. Observation of the kinetics of phagocytosis inhibition ( Fig. 2b,d ), which was significant after 60 min of Tat uptake only and plateaued after 3–4 h, was consistent with this interpretation. We examined Tat endocytosis by MDMs using immunofluorescence. Fluorescent transferrin and anti-Lamp-1 antibodies were used to localize early and late endosomal structures, respectively [19] . Tat was prebound at 4 °C before washes and cell incubation at 37 °C to allow synchronous uptake. Representative images (after 60 min of endocytosis) are shown in Fig. 3a together with the efficiency of co-localization with endocytic markers calculated using Manders’ coefficient ( Fig. 3b ). The co-localization of Tat or Tat-W11Y with transferrin and especially Lamp-1 increased with time and peaked at ~45 min. After this time, Tat co-localization with Lamp-1 strongly decreased, while that of Tat-W11Y with Lamp-1 remained stable. These results are consistent with the identification of late endosomes as the elements of the endocytic pathway from which Tat escapes to reach the cytosol [19] , and the inability of Tat-W11Y to escape from endosomes [18] . The kinetics of Tat intracellular transport in MDMs is consistent with those of phagocytosis inhibition ( Fig. 2b,d ) and indicates that Tat, but not Tat-W11Y, rapidly escapes to the cytosol to affect the phagocytic machinery. 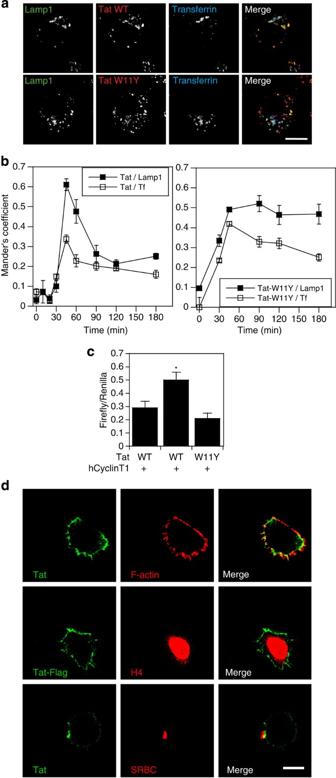Figure 3: Internalization of HIV-1 Tat by human macrophages. (a) Human MDMs were labelled with Tat or Tat-W11Y on ice, washed at 4 °C and then incubated at 37 °C for 60 min. Transferrin-Cy5 was added for the last 40 min. Cells were then processed for detection of Tat and Lamp-1 by immunofluorescence, before examination under a confocal microscope. Representative median optical sections are shown. Scale bar, 10 μm. (b) MDMs were allowed to internalize Tat for different times. Co-localization between the different tracers was quantified using the Mander’s coefficient (mean±s.e.m. withn=3). (c) Mouse RAW 264.7 macrophages were cotransfected with pGL3-LTR and pRL-TK that contain a Firefly or Renilla luciferase gene under the control of HIV-1 LTR or thymidine kinase, respectively. When indicated, a human cyclin T1 vector was added to enable transactivation by Tat since mouse cyclin T1 does not efficiently support this process61. Tat was added after 18 h and luciferase activities were assayed 24 h later. Transactivation was monitored as the increase in the Firefly/Renilla luciferase activity ratio. Results (mean±s.e.m.) from a typical experiment withn=3. Student’st-test was performed between the ±cyclin T conditions (*P<0.05). (d) RAW 264.7 macrophages were transfected with Tat or Tat-Flag. After 24 h, cells were fixed and Tat, Flag or histone H4 were labelled using antibodies while F-actin was stained using fluorescent phalloidin. When indicated, IgG-opsonized SRBCs were added to cells for 3 min at 37 °C before fixation. Median confocal sections are shown. Scale bar, 10 μm. Figure 3: Internalization of HIV-1 Tat by human macrophages. ( a ) Human MDMs were labelled with Tat or Tat-W11Y on ice, washed at 4 °C and then incubated at 37 °C for 60 min. Transferrin-Cy5 was added for the last 40 min. Cells were then processed for detection of Tat and Lamp-1 by immunofluorescence, before examination under a confocal microscope. Representative median optical sections are shown. Scale bar, 10 μm. ( b ) MDMs were allowed to internalize Tat for different times. Co-localization between the different tracers was quantified using the Mander’s coefficient (mean±s.e.m. with n =3). ( c ) Mouse RAW 264.7 macrophages were cotransfected with pGL3-LTR and pRL-TK that contain a Firefly or Renilla luciferase gene under the control of HIV-1 LTR or thymidine kinase, respectively. When indicated, a human cyclin T1 vector was added to enable transactivation by Tat since mouse cyclin T1 does not efficiently support this process [61] . Tat was added after 18 h and luciferase activities were assayed 24 h later. Transactivation was monitored as the increase in the Firefly/Renilla luciferase activity ratio. Results (mean±s.e.m.) from a typical experiment with n =3. Student’s t -test was performed between the ±cyclin T conditions (* P <0.05). ( d ) RAW 264.7 macrophages were transfected with Tat or Tat-Flag. After 24 h, cells were fixed and Tat, Flag or histone H4 were labelled using antibodies while F-actin was stained using fluorescent phalloidin. When indicated, IgG-opsonized SRBCs were added to cells for 3 min at 37 °C before fixation. Median confocal sections are shown. Scale bar, 10 μm. Full size image To examine whether Tat is actually delivered to the cytosol following endocytosis, we used a transactivation assay. We transfected mouse RAW 264.7 macrophages with luciferase reporter plasmids; human cyclin T1 was cotransfected because mouse cyclin T1 only enables weak transactivation activity [32] . Following the addition of recombinant Tat to the medium, we found that WT Tat was able to transactivate in a cyclin T1-dependent manner ( Fig. 3c ), while this was not the case for Tat-W11Y. Hence, extracellular Tat can reach the macrophage cytosol. Tat is recruited to the phagocytic cup To examine the intracellular localization of Tat in macrophages, we transiently expressed Tat within RAW 264.7 macrophages whose phagocytic activity has been extensively characterized [33] , [34] , [35] . As previously observed in primary CD4 + T cells [14] , transfected Tat concentrated at the plasma membrane of RAW macrophages ( Fig. 3d ). When Tat-transfected cells were stained both for Tat and histone H4, a strong histone labelling was observed in the nucleus, while Tat was only detected at the plasmalemma, confirming that this localization was not due to a poor permeabilization of the nuclear envelope during immunofluorescence processing. Tat mutants unable to bind PI(4,5)P2 (Tat-W11Y and Tat (49–51)A) were essentially cytosolic, while a control mutant (Tat (55–57)A) was still membrane bound ( Supplementary Fig. 4 ). Hence, PI(4,5)P 2 is responsible for Tat localization to the macrophage plasmalemma. PI(4,5)P 2 binding enables Tat to inhibit phagocytosis PI(4,5)P 2 is concentrated at the phagocytic cup during FcγR-mediated phagocytosis [33] , and we found that Tat was recruited to the phagocytic cup on interaction of Tat-transfected macrophages with IgG-opsonized sheep red blood cells (SRBCs; Fig. 3d ), suggesting that Tat interacts with PI(4,5)P 2 at this level. To examine whether Tat binding to PI(4,5)P 2 is required for Tat to inhibit phagocytosis, we used Tat(49–51)A and Tat-W11Y that do not bind PI(4,5)P 2 (ref. 14 ). None of these mutants caused inhibition of FcγR-mediated or MR-mediated phagocytosis, while the control mutant Tat(55–57)A was as effective as Tat ( Fig. 4a ). To confirm that phagocytosis inhibition requires Tat-PI(4,5)P 2 interaction we tried to increase cellular PI(4,5)P 2 levels by expressing the major PI(4,5)P 2 synthesizing enzymes, that is, PIP kinases α or β [36] (haemagglutinin (HA) tagged) into RAW 264.7 macrophages. We first examined by immunofluorescence whether the enzymes were indeed expressed and if their expression induced an increase in PI(4,5)P 2 levels. PIPKiα was observed diffused in the cytosol while PIPKiβ was more at the plasma membrane ( Fig. 4b ). When PI(4,5)P 2 was detected using the 2C11 monoclonal antibody it was found at the plasmalemma, and enzyme overexpression lead to a significant increase in PI(4,5)P 2 level, especially for PIPKiβ (+450%; Fig. 4b ). This overexpression had no effect on phagocytosis efficiency ( Fig. 4c ), indicating that PI(4,5)P 2 is not limiting for phagocytosis. Nevertheless, on enzyme cotransfection with Tat, PIPKis prevented Tat to affect FcγR- or MR-mediated phagocytosis ( Fig. 4c ). Collectively these data show that phagocytosis inhibition results from Tat binding to PI(4,5)P 2 . This interaction apparently disorganizes the phagocytosis machinery, probably by affecting the recruitment of one of its key components. It is noteworthy that the absence of effect of transfected Tat-W11Y, which transactivates LTR-driven genes as efficiently as WT Tat on transfection into cells [18] , shows that the transcriptional activity of Tat is not involved in its capacity to inhibit phagocytosis. 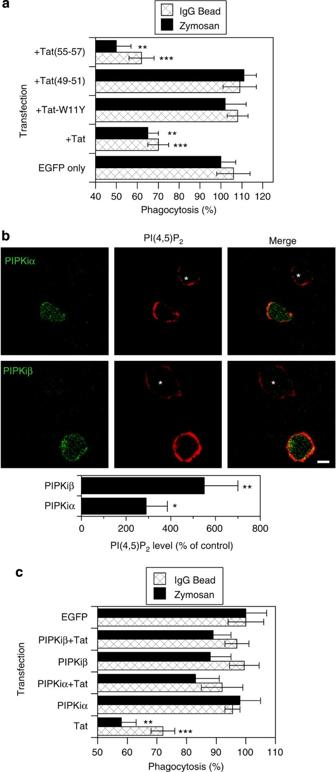Figure 4: PI(4,5)P2binding is required for Tat to inhibit phagocytosis. (a) RAW 264.7 macrophages were transfected with a vector encoding EGFP alone (control cells) or EGFP and the indicated Tat mutant. Tat-W11Y and Tat(49–51)A are unable to bind PI(4,5)P2, while the control mutant Tat(55–57)A does14. After 24 h, the macrophages were allowed to phagocytose IgG-coated beads or zymosan, before labelling extracellular particles on ice and counting using a fluorescent microscope. Data are mean±s.e.m. of three independent experiments. (b) Cells were transfected with HA-tagged PIPKi α or β as indicated. After 24 h, macrophages were fixed and processed for anti-PI(4,5)P2and anti-HA immunofluorescence60before viewing under a confocal microscope. Median optical sections are shown. Control cells are indicated by a star. Scale bar, 5 μm. The graph shows the quantification of the PI(4,5)P2fluorescence level (mean±s.e.m.) fromn>20 cells. (c) The vector encoding EGFP and Tat was cotransfected (ratio 1/1) with an empty vector or with an expression vector for the indicated isoform of PIPKi before assaying phagocytosis of IgG-coated beads or Zymosan. Data are mean±s.e.m. of three independent experiments and Student’st-test (***P<0.001; **P<0.01, *P<0.05) were performed comparing with the transfection control. EGFP transfection did not significantly affect phagocytosis efficiency or PI(4,5)P2levels. Figure 4: PI(4,5)P 2 binding is required for Tat to inhibit phagocytosis. ( a ) RAW 264.7 macrophages were transfected with a vector encoding EGFP alone (control cells) or EGFP and the indicated Tat mutant. Tat-W11Y and Tat(49–51)A are unable to bind PI(4,5)P 2 , while the control mutant Tat(55–57)A does [14] . After 24 h, the macrophages were allowed to phagocytose IgG-coated beads or zymosan, before labelling extracellular particles on ice and counting using a fluorescent microscope. Data are mean±s.e.m. of three independent experiments. ( b ) Cells were transfected with HA-tagged PIPKi α or β as indicated. After 24 h, macrophages were fixed and processed for anti-PI(4,5)P 2 and anti-HA immunofluorescence [60] before viewing under a confocal microscope. Median optical sections are shown. Control cells are indicated by a star. Scale bar, 5 μm. The graph shows the quantification of the PI(4,5)P 2 fluorescence level (mean±s.e.m.) from n >20 cells. ( c ) The vector encoding EGFP and Tat was cotransfected (ratio 1/1) with an empty vector or with an expression vector for the indicated isoform of PIPKi before assaying phagocytosis of IgG-coated beads or Zymosan. Data are mean±s.e.m. of three independent experiments and Student’s t -test (*** P <0.001; ** P <0.01, * P <0.05) were performed comparing with the transfection control. EGFP transfection did not significantly affect phagocytosis efficiency or PI(4,5)P 2 levels. Full size image Phagocytosis inhibition by Tat involves Cdc42 The similarity of dose/response curves for FcγR- and MR-mediated phagocytosis ( Fig. 2a,c ) indicated that Tat target might be the same in both pathways, but not involved in complement-mediated phagocytosis. We thus focused on Cdc42, which is involved in both pathways [1] , [3] , and whose recruitment at the phagocytic cup relies on PI(4,5)P 2 (refs 1 , 37 ). As observed earlier [38] , [39] , [40] , dominant negative (DN) versions of Cdc42 and Rac1 potently inhibit FcγR-mediated phagocytosis but, on cotranfection with Tat, DN-Rac1 only showed synergistic inhibition, indicating that Tat affects Cdc42- but not Rac1-pathway ( Fig. 5a ). The use of short interfering RNAs (siRNAs) against Rac1 or Cdc42 that potently inhibit the expression of their respective target ( Fig. 5b ) provided similar data ( Fig. 5a ). When zymosan phagocytosis was assayed, we also observed that Tat did not synergize with DN-Cdc42 or siRNA against Cdc42 ( Fig. 5c ). As observed before [3] , we did not find MR-mediated phagocytosis to rely on Rac1 ( Fig. 5c ). 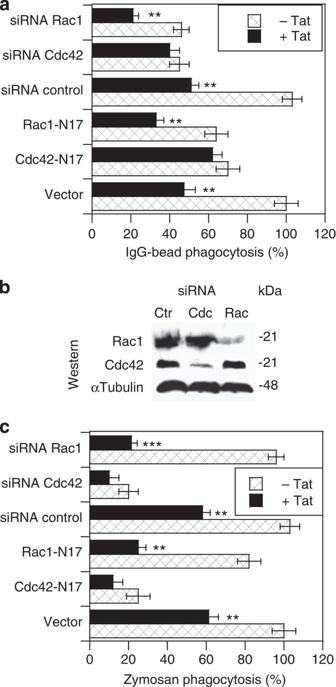Figure 5: Phagocytosis inhibition by Tat involves Cdc42. RAW 264.7 macrophages were cotransfected (1/1) with a DN (N17) GTPase and a Tat-encoding or empty vector or with Tat and the indicated siRNA. (a) Phagocytosis of IgG-opsonized beads was assayed after 24 h. A minimum of 60 transfected cells (identified using EGFP fluorescence) were imaged. (b) Cells were plated in six-well plates before transfection with siRNA control (Ctr), against Cdc42 (Cdc) or Rac1 (Rac). Cells were lysed before western blotting against Rac1, Cdc42 or α tubulin as a loading control. (c) Cells were transfected as inabefore assaying zymosan phagocytosis. Data are mean±s.e.m. of three independent experiments and Student’st-test (***P<0.001; **P<0.01) were performed comparing with the minus Tat conditions. Figure 5: Phagocytosis inhibition by Tat involves Cdc42. RAW 264.7 macrophages were cotransfected (1/1) with a DN (N17) GTPase and a Tat-encoding or empty vector or with Tat and the indicated siRNA. ( a ) Phagocytosis of IgG-opsonized beads was assayed after 24 h. A minimum of 60 transfected cells (identified using EGFP fluorescence) were imaged. ( b ) Cells were plated in six-well plates before transfection with siRNA control (Ctr), against Cdc42 (Cdc) or Rac1 (Rac). Cells were lysed before western blotting against Rac1, Cdc42 or α tubulin as a loading control. ( c ) Cells were transfected as in a before assaying zymosan phagocytosis. Data are mean±s.e.m. of three independent experiments and Student’s t -test (*** P <0.001; ** P <0.01) were performed comparing with the minus Tat conditions. Full size image Tat prevents the recruitment of Cdc42 to the phagocytic cup To obtain more direct evidence for the implication of Cdc42 in Tat effect, we examined whether exogenous Tat affected the recruitment of green fluorescent protein (GFP)-tagged GTPases at the phagocytic cup, first during FcγR-mediated phagocytosis of opsonized SRBCs. As observed earlier [1] , in >80% of the cells Cdc42 is recruited to the rims of the cup ( Fig. 6a ), where PI(4,5)P 2 accumulates ( Supplementary Fig. 5 ). We found that in ~85% of the cells Tat prevented the recruitment of Cdc42 that remained largely cytosolic, while Rac1 recruitment to the cup remained unaffected ( Fig. 6a,b ). In agreement with functional assays ( Fig. 5a ), recruitment of Cdc42 to the cup was insensitive to Tat-W11Y and the overexpression of PIPKi β prevented Tat to affect Cdc42 recruitment to the cup ( Fig. 6a,b ). Identical data were obtained when Tat was applied intracellularly (that is, transfected, Supplementary Fig. 6 ), when zymosan was used as a phagocytic target ( Supplementary Fig. 7 ), or when living cells were used ( Supplementary Fig. 8 ; Supplementary Movies 1 and 2 ). Altogether these data show that Tat inhibits phagocytosis by preventing Cdc42 recruitment to the cup, thereby impairing this key GTPase to fulfil its role at this level. 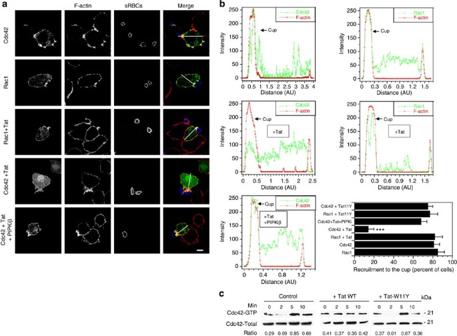Figure 6: Tat prevents Cdc42 recruitment to the phagocytic cup and its subsequent activation. (a) RAW 264.7 macrophages were transfected with a vector encoding the indicated EGFP-GTPase chimera. When indicated, PIPKiβ was cotransfected (ratio 1/1). After 18 h, cells were treated with 10 nM Tat or Tat-W11Y for 5 h before adding IgG-opsonized SRBCs for 3 min, fixation, permeabilization, F-actin staining using fluorescent phalloidin and SRBCs labelling with fluorescent antibodies. Cells were viewed under a confocal microscope. Scale bar, 5 μm. (b) Line plots (width: five pixels) indicated on the merged images were generated to follow signal accumulation in the phagocytic cup. The histogram shows the percentage of cells (with one cup) displaying significant accumulation at the cup (mean±s.e.m. withn>20 cells). Student’st-test (***P<0.001) was performed comparing with the minus Tat conditions. (c) GTPase activation assay. RAW 264.7 macrophages were pretreated or not with Tat (WT or W11Y) for 5 h. IgG-opsonized SRBCs were then added to macrophages for the indicated times before lysing cells and pulling-down activated Cdc42. Pulled-down and total Cdc42 were analysed by Western blot. Bands were quantified to determine the activated/total Cdc42 ratio. One representative experiment of three is shown. Figure 6: Tat prevents Cdc42 recruitment to the phagocytic cup and its subsequent activation. ( a ) RAW 264.7 macrophages were transfected with a vector encoding the indicated EGFP-GTPase chimera. When indicated, PIPKiβ was cotransfected (ratio 1/1). After 18 h, cells were treated with 10 nM Tat or Tat-W11Y for 5 h before adding IgG-opsonized SRBCs for 3 min, fixation, permeabilization, F-actin staining using fluorescent phalloidin and SRBCs labelling with fluorescent antibodies. Cells were viewed under a confocal microscope. Scale bar, 5 μm. ( b ) Line plots (width: five pixels) indicated on the merged images were generated to follow signal accumulation in the phagocytic cup. The histogram shows the percentage of cells (with one cup) displaying significant accumulation at the cup (mean±s.e.m. with n >20 cells). Student’s t -test (*** P <0.001) was performed comparing with the minus Tat conditions. ( c ) GTPase activation assay. RAW 264.7 macrophages were pretreated or not with Tat (WT or W11Y) for 5 h. IgG-opsonized SRBCs were then added to macrophages for the indicated times before lysing cells and pulling-down activated Cdc42. Pulled-down and total Cdc42 were analysed by Western blot. Bands were quantified to determine the activated/total Cdc42 ratio. One representative experiment of three is shown. Full size image Tat does not affect PI(3,4,5)P 3 -mediated recruitment We then checked whether Tat could interfere with late phagocytosis stages. Following the increase of PI(4,5)P 2 at the cup, it is depleted with a concomitant increase in PI(3,4,5)P 3 that persists until the phagosome closure [1] . We thus used a GFP chimera of PH Akt that tightly binds to PI(3,4,5)P 3 (ref. 14 ) to examine whether Tat could affect PI(3,4,5)P 3 production at the cup and/or perturb the recruitment of effectors by this phosphoinositide. In agreement with the poor affinity of Tat for PI(3,4,5)P 3 (ref 14 ), we did not find that cotransfected Tat significantly affected the recruitment to the cup of PH Akt ( Supplementary Fig. 9 ). Hence, Tat does not interfere with PI(3,4,5)P 3 -dependent steps of phagocytosis. Tat prevents Cdc42 activation by IgG-opsonized targets The recruitment of Rho GTPases at the plasma membrane takes place before their activation by guanine nucleotide exchange factors that stimulate the exchange of GDP for GTP to generate the active form of the GTPase that is capable of interacting with downstream effectors and targets [41] . Since Tat prevents the recruitment of Cdc42 at the phagocytic cup, it should thus inhibit Cdc42 activation. To examine this point, we first used a biochemical GTPase activation assay that is based on the interaction of Cdc42 with the Cdc42-binding domain (CRIB) from human PAK1B coupled to GST [42] . For both control and Tat-W11Y pretreated macrophages a strong activation of Cdc42 was detected 5 min after adding IgG-coated SRBCs to control RAW 264.7 macrophages. Nevertheless, no Cdc42 activation was detected for WT Tat pretreated macrophages ( Fig. 6c ). To confirm this data, we monitored Cdc42 activation in living cells using the Raichu Cdc42 probe and fluorescence resonance energy transfer (FRET) [43] . As observed earlier [44] , we found that macrophage contact with an opsonized target induces a strong Cdc42 activation at the cup, while when macrophages were pretreated with Tat no Cdc42 activation was observed at the cup ( Supplementary Fig. 8 ; Supplementary Movies 1 and 2 ). Collectively, these data show that Tat prevents the recruitment and activation of Cdc42 at the phagocytic cup. Tat is a strong inhibitor of Cdc42 We then compared the efficiency of phagocytosis inhibition by Tat and a specific Cdc42 inhibitor, ML-141 (also termed CID2950007) [45] . Neither ML-141 nor Tat significantly affected CR3-mediated phagocytosis ( Fig. 7a ). Tat was as effective as ML-141 in inhibiting the phagocytosis of IgG beads or zymosan ( Fig. 7a ) as well as in preventing the uptake of M. avium or opsonized Toxoplasma ( Fig. 7b ). These results show that Tat is a strong Cdc42 inhibitor. They also confirm that Cdc42 is needed for FcγR- and MR- but not complement-mediated phagocytosis in MDMs. 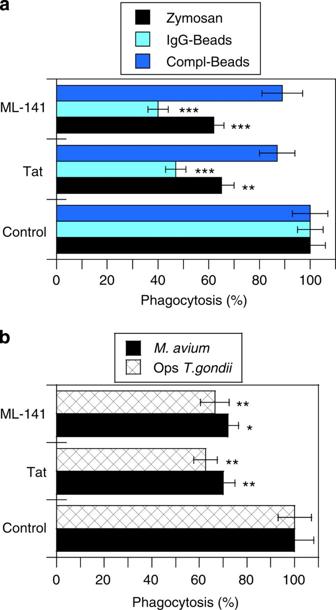Figure 7: Tat is a strong Cdc42 inhibitor. MDMs were treated with 2 nM Tat or 10 μM ML-141 for 5 h before assaying phagocytosis of (a) IgG beads, fluorescent zymosan or C3bi-coated beads (compl-beads) or (b)M. aviumor opsonizedT. gondii. Data are mean±s.e.m. of three independent experiments. Phagocytosis of unopsonizedT. gondiiwas negligible (~6% of opsonized control). Student’st-test (***P<0.001; **P<0.01; *P<0.05) were performed comparing with the control conditions. Figure 7: Tat is a strong Cdc42 inhibitor. MDMs were treated with 2 nM Tat or 10 μM ML-141 for 5 h before assaying phagocytosis of ( a ) IgG beads, fluorescent zymosan or C3bi-coated beads (compl-beads) or ( b ) M. avium or opsonized T. gondii . Data are mean±s.e.m. of three independent experiments. Phagocytosis of unopsonized T. gondii was negligible (~6% of opsonized control). Student’s t -test (*** P <0.001; ** P <0.01; * P <0.05) were performed comparing with the control conditions. Full size image Tat inhibits pseudopod elongation To further confirm that Tat prevents Cdc42 action during phagocytosis, and to examine the morphological consequences of this inhibition, we first used scanning electron microscopy (SEM). Indeed, the inactivation of Cd42 function during FcγR phagocytosis is known to promote the accumulation of cups with short pseudopods [38] . Accordingly, on observation by SEM of MDMs that have been pretreated with ML-141 before adding IgG-coated beads, macrophages accumulate such intermediates, that is, beads incompletely covered by pseudopods. This was the case for ~60% of the beads. These intermediates were observed in the same proportions following Tat pretreatment, while the vast majority of control cells (not treated or treated with Tat-W11Y) showed beads entirely engulfed (75–85% of the beads; Fig. 8a,b ). Similar results were obtained using zymosan as phagocytic target ( Supplementary Fig. 10 ). To obtain quantitative data, we measured pseudopod length using IgG-coated 3 μm beads, phalloidin-labelled macrophages and confocal sections centred on the equatorial plane of the beads. We found that Tat significantly reduced the pseudopod length by ~25%, while Tat-W11Y had no effect ( Fig. 8c,d ). 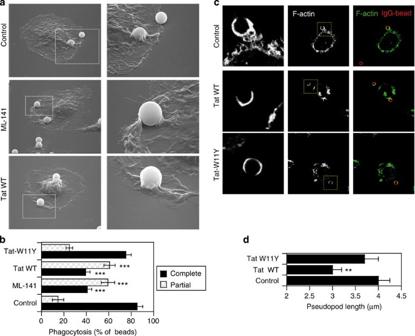Figure 8: Tat impairs pseudopod elongation during phagocytosis. (a) Human MDMs were treated with 10 μM ML-141 or 2 nM Tat or Tat-W11Y for 5 h before adding IgG-opsonized beads for 3 min, fixation and processing for SEM. Beads are 3 μm in diameter. The right panels are magnifications of boxed regions in the left panels. (b) The histogram shows the percentage of beads (mean±s.e.m.,n=3 independent experiments with >30 beads counted for each) that were entirely or partially engulfed under each condition. (c) MDMs were pretreated with Tat or Tat-W11Y before adding IgG-opsonized beads for 3 min, fixation, permeabilization, staining beads with fluorescent antibodies and F-actin with fluorescent phalloidin. Confocal sections (~0.8-μm thick) were centred on the equatorial plane of the bead. The left panels are magnifications of boxed regions in the central panels. (d) Fifty cups were imaged for each condition and pseudopod length (±s.e.m.) was measured using imageJ. Student’st-test (***P<0.001; **P<0.01) were performed comparing with the control conditions. Figure 8: Tat impairs pseudopod elongation during phagocytosis. ( a ) Human MDMs were treated with 10 μM ML-141 or 2 nM Tat or Tat-W11Y for 5 h before adding IgG-opsonized beads for 3 min, fixation and processing for SEM. Beads are 3 μm in diameter. The right panels are magnifications of boxed regions in the left panels. ( b ) The histogram shows the percentage of beads (mean±s.e.m., n =3 independent experiments with >30 beads counted for each) that were entirely or partially engulfed under each condition. ( c ) MDMs were pretreated with Tat or Tat-W11Y before adding IgG-opsonized beads for 3 min, fixation, permeabilization, staining beads with fluorescent antibodies and F-actin with fluorescent phalloidin. Confocal sections (~0.8-μm thick) were centred on the equatorial plane of the bead. The left panels are magnifications of boxed regions in the central panels. ( d ) Fifty cups were imaged for each condition and pseudopod length (±s.e.m.) was measured using imageJ. Student’s t -test (*** P <0.001; ** P <0.01) were performed comparing with the control conditions. Full size image It is well established that the phagocytic function of neutrophils and cells of the macrophage lineage is impaired in HIV-1-infected patients [8] , [9] , [12] , [13] . Both FcγR- and MR-mediated phagocytosis are inhibited, enabling the development of several opportunistic pathogens [12] , [46] . More contrasted results were obtained for CR3-mediated phagocytosis, and it is therefore unclear whether this pathway is affected following HIV-1 infection [47] , [48] . It should be noted that most of these pioneer studies did not score phagocytosis separately in infected and bystander macrophages. Nevertheless, because >90% of monocytes and macrophages are uninfected in patients [8] , [9] , [12] , these observations indicated that uninfected macrophages are also affected in their capacity to perform FcγR- and MR-mediated phagocytosis. Such a bystander effect of HIV-1 infection on uninfected macrophages was indeed detected in vitro when monitoring FcγR-mediated phagocytosis [24] , but the underlying mechanism remained elusive. Several studies nevertheless showed that HIV-1 infection does not significantly affect the surface expression of phagocytic receptors, indicating that the inhibition of phagocytosis by HIV-1 occurs after the receptor recognition step [12] . It has also been observed that Cdc42 failed to be activated following zymosan addition to HIV-1-infected macrophages but, again, it was unclear whether this was due to infected and/or bystander cells and what was the underlying mechanism [3] . Here, we found that phagocytosis inhibition in bystander neutrophils, monocytes and macrophages is due to secreted HIV-1 Tat that efficiently inhibits this process at subnanomolar concentration. This protein is known to be actively secreted by infected cells [14] , [49] and is present at nanomolar concentration in the sera of HIV-1 infected patients [15] , [16] . It still seems to be present in the sera of HIV-1 patients under antiretroviral therapy [50] . The role of circulating Tat in progression to AIDS is also suggested by the correlation observed between the presence of anti-Tat antibodies and non-progression to AIDS [51] , even if these antibodies are poorly neutralizing [50] . In agreement with clinical data indicating that these pathways are specifically affected in HIV-1-infected patients [12] , [46] , we found that Tat inhibits both FcγR- and MR-mediated phagocytosis in macrophages. Moreover, Tat inhibited FcγR-mediated phagocytosis in human monocytes and neutrophils, phagocytes that do not express significant amounts of the MR [25] . We did not observe any significant effect of Tat on CR3-mediated phagocytosis. The capacity of Tat to reach the cell cytosol from the outside is well documented [17] , and we found that Tat needs to enter macrophages to affect MR- and FcγR-mediated phagocytosis. On cytosolic delivery Tat binds PI(4,5)P 2 at the phagocytic cup. This interaction is necessary and sufficient for Tat to inhibit phagocytosis. Phosphoinositides such PI(4,5)P 2 and/or PI(3,4,5)P 3 enable the recruitment to the plasma membrane of small GTPases such as Cdc42 and Rac1 (ref. 6 ) that are master regulators of actin polymerization during phagocytosis [1] . The place and timing of phosphoinositide enrichment at the phagocytic cup is tightly regulated. PI(4,5)P 2 is concentrated at the rims of the cup at the beginning of the cup formation, before its depletion. This disappearance of PI(4,5)P 2 is concomitant with the enrichment of the entire cup in PI(3,4,5)P 3 that persists until after the phagosome seals [1] , [33] . Interestingly, these localizations and kinetics parallel those of GTPase recruitment and activation since Cdc42 activation specifically takes place at the rims of the cup before Rac1 activation that occurs throughout the phagocytic cup [44] . These temporal and spatial correlations suggest that Cdc42 and Rac1 recruitment and activation specifically rely on PI(4,5)P 2 and PI(3,4,5)P 3 , respectively. Moreover, isoprenylated Cdc42 was found to bind directly and tightly to liposomes as long as they contain PI(4,5)P 2 (ref. 37 ). We found accordingly that Tat, which binds PI(4,5)P 2 with a very high affinity but not significantly PI(3,4,5)P 3 (ref. 14 ), prevents the recruitment of Cdc42 at the cup without affecting the recruitment of Rac1 or of PH Akt , a well-characterized PI(3,4,5)P 3 ligand [14] . Tat thereby inhibits the first phase of pseudopod elongation, which is under the control of Cdc42 (ref. 38 ) and independent of class-I PI 3-Kinase, but not the second phase that requires PI(3,4,5)P 3 (ref. 52 ). Hence, when PI(4,5)P 2 is made available at the cup for Cdc42, if Tat is present it binds to this lipid and thereby prevents Cdc42 recruitment and activation. All PI(4,5)P 2 molecules present within the cell are probably not all available for Tat and Cdc42 and Tat does not have to titrate the entire cellular pool of PI(4,5)P 2 to generate an effect, just a subset. Accordingly, when the cell is forced to make more PI(4,5)P 2 by PIPKi overexpression, Tat is diluted among these PI(4,5)P 2 molecules, Cdc42 recruitment is restored and phagocytosis proceeds normally. The identification of Cdc42 as Tat target in the phagocytic machinery is consistent with its capacity to perturb FcγR- and MR- but not CR3-mediated phagocytosis, since Cdc42 is the only regulating GTPase that is required for FcγR- and MR- but not for CR3-phagocytosis pathway [1] , [2] , [3] . Small GTPases of the Rho superfamily are key regulators of phagocytosis and the targets of several bacterial toxins that can activate or inhibit these key effectors by proteolysis, post-translational modifications or by mimicking host Rho regulators [53] . Tat is an original toxin in this field since it affects Cdc42 function by preventing its recruitment to the phagocytic cup, thereby preventing its activation. Hence, Tat is a PI(4,5)P 2 targeting toxin that can affect the neurosecretory [54] , the phagocytic (this study) and probably other PI(4,5)P 2 -dependent membrane traffic machineries. It should be noted that Tat targets in these biological systems are different, Annexin A2 (ref. 54 ) for neurons/exocytosis and Cdc42 (this study) for macrophages/phagocytosis. The capacity of Tat to perturb these activities is also different since subnanomolar concentrations of Tat are sufficient to efficiently inhibit phagocytosis, while 5–10 nM of Tat are required to affect the neurosecretory activity [54] . The phagocytic machinery thus seems to be a preferential target of circulating Tat. Why isn’t Tat able to inhibit phagocytosis in infected cells? We found that the virus sets up a system to promote a very efficient secretion of Tat from infected cells while Tat remains on PI(4,5)P 2 in target cells (Chopard et al ., manuscript in preparation). This result is consistent with the finding that Nef, which is not secreted by infected cells [14] , is responsible for phagocytosis inhibition in infected cells [55] . The virus, therefore, uses two different proteins to effectively inhibit phagocytosis in infected and uninfected macrophages. We thus provided here biochemical, functional and morphological evidence that Tat, at the minute doses observed in the sera of HIV-1-infected patients potently inhibits PI(4,5)P 2 -mediated Cdc42 recruitment and activation to the phagocytic site in macrophages. Tat thereby affects pseudopod elongation impairing the FcγR- and MR-mediated phagocytosis of opportunistic pathogens and favouring their multiplication. Since Tat also inhibits FcγR-mediated phagocytosis in monocytes and neutrophils, these data provide a molecular basis for the global phagocytic defect of a wide range of phagocytes following HIV-1 infection. Reagents All cell lines were obtained from the American Tissue Culture Collection, except the Jurkat CD4-CCR5 cell line that was from the centre for AIDS reagents (NIBSC, UK). Rabbit anti-SRBCs, polystyrene beads (LB30, 3 μm diameter), zymosan A, fluorescein isothiocyanate (FITC), fluorescent phalloidins and anti-FlagM2 were from Sigma. SRBCs were from Eurobio or Sordalab. The Cdc42 inhibitor ML-141 was from Tocris and was used at 10 μM (ref. 45 ). Rabbit anti-Tat (HXB2) antibodies were obtained from Erwann Loret (Marseille, France), rabbit anti-histone H4 antibodies were from Serotec (#AHP413), rabbit anti-Lamp-1 from Abcam (#24170), anti-zymosan from Life Technologies (#Z2850), anti- M. avium from Serotec (#63970506), anti-Cdc42 (#PA1-0192) and anti-Rac1 (#PA1-0191) from Thermo, fluorescein-antiCD206 (#551135), fluorescein-antiCD64 (#555527) and isotypic control (#555909) from BD biosciences, and anti-HA tag (high affinity; #1867423) from Roche. The 2C11 antiPI(4,5)P 2 monoclonal IgMs were from Abcam (#11039). Anti-HIV-1 p24 for immunofluorescence and fluorescence-activated cell sorting (FACS) were from AIDS reagents (#6457) and Beckman-Coulter (Kc57- fluorescein; #CO6604665), respectively. Anti T. gondii human serum was kindly provided by J.F. Dubremetz [56] . Secondary antibodies were from Jackson ImmunoResearch. Transferrin was labelled with Cy5 as recommended by the manufacturer (GE Healthcare). Mission siRNAs against mouse Cdc42 (5′- CAAAUUCCCAUCGGAAUAU -3′) and rac1 (5′- CACCUAAGCACUAAACUCU -3′) were from Sigma. HIV-1 virions were produced by first transfecting 293T cells. The transfection supernatants were then used to infect Jurkat CD4-CCR5 cells to obtain higher viral titres. The viral concentration was monitored by Gag p24 ELISA assay (Innotest, Ingen, France) [14] . Lipofectamine 2000, Lipofectamine 3000 and RNAiMAX were from Life Technologies. The GST chimera of the CRIB from human PAK1B (amino acids 56–272) was produced in Escherichia coli BL21 cells as described [42] . In brief, bacteria were induced for 3 h and then lysed in 150 mM NaCl, 5 mM MgCl 2 , 1 mM dithiothreitol, 50 mM Tris, pH 7.5 supplemented with 0.5% Triton-X-100 and antiproteases (Complete, Roche). Following sonication, the lysate was centrifuged at 4 °C for 30 min at 20,000 g. Glutathione-agarose was then added to the supernatant, before incubation for 1 h at 4 °C on a rotating wheel. Beads were then washed with lysis buffer and stored at −80 °C in lysis buffer supplemented with 10% glycerol. Plasmids and cell transfection or infection Tat (BH10 isolate, 86 residues) and Tat-Flag were cloned into pBi (Clontech) for expression in mammalian cells [14] . This bicistronic vector independently encodes EGFP and Tat. Vectors for HA-tagged PIPKi α and β were from Gregory Longmore, Cdc42 Raichu probe from Stephane Bodin, Rac1-GFP and Cdc42-GFP from Cecile Gauthier-Rouvière, Rac1-N17 and Cdc42-N17 from Delphine Muriaux, PH Akt -EGFP from Georges Bismuth, 5-phosphatase IV from Akira Ono and pcDNA-human cyclin T1 from Rosemary Kiernan. RAW 264.7 mouse macrophages were obtained and cultured according to the recommendations of the American Tissue Culture Collection. They were transfected with plasmids (±siRNA) using Lipofectamine 2000 or 3000 as recommended by the manufacturer. For siRNA transfection, cells were transfected twice using RNAiMAX with a 24-h interval and were harvested after 48 h. For the preparation of human monocytes, neutrophils and MDMs, freshly drawn human blood was obtained from the local blood bank (Etablissement Français du Sang, Montpellier). Peripheral blood mononuclear cells were prepared by density gradient separation on Ficoll–Hypaque (Eurobio). Monocytes and CD4+ T cells were then purified using CD14 microbeads (Miltenyi Biotec’s) and a CD4 Easysep Negative Selection Kit (Stemcell), respectively. Monocytes were then matured to macrophages by cultivation for 6–8 days in the presence of 50 ng ml −1 macrophage colony-stimulating factor (Immunotools), before infection by HIV-1 (Ad8; multiplicity of infection=0.5). T cells were activated using phytohemagglutinin (1 μg ml −1 ) for 24 h then interleukin-2 (50 U ml −1 ) for 6 days before infection by HIV-1 (NL4-3; multiplicity of infection=0.5) (ref. 14 ). After 24 h, control or infected T cells were washed and then added to Transwells (0.4 μm pore size) in 24-well plates containing macrophages (10 T-cells per macrophage) on coverslips. Cells were cocultured for 8–9 days before assaying IgG-bead phagocytosis. Infection was monitored using p24-immunofluorescence for macrophages, together with p24 enzyme-linked immunosorbent assay. For T cells, infection was monitored using intracellular FACS analysis [14] . To this end, cells were fixed with 2% paraformaldehyde in PBS for 20 min, washed with PBS supplemented with 1% fetal bovine serum (PBS/FBS) then resuspended in permeabilization buffer (PBS supplemented with 1% FBS, 5 mM EDTA and 0.2% saponin). After 10 min, cells were centrifuged (2 min × 2,000 g ) then resuspended in Kc57-Fluorescein (or an isotypic control) diluted 1/100 in permeabilization buffer. After 30 min, cells were washed once with PBS/FBS then with PBS. They were finally postfixed with 1% paraformaldehyde in PBS before FACS analysis on a FACScalibur (Becton Dickinson). Tat concentration in macrophage supernatants was evaluated by western blotting. Neutrophils were prepared essentially as described [57] . In brief, following the Ficoll–Hypaque gradient, the erythrocyte–granulocyte pellets were resuspended in ice-cold H 2 O for 30 s to lyse the erythrocytes. Isotonicity was restored with 10 × HBSS (Hank’s balanced salt solution), cells were pelleted for 10 min at 200 g and the lysis was repeated using 0.2% NaCl instead of H 2 O. The resulting polymorphonuclear cells were then loaded on a discontinuous 70/60% Percoll gradient that was centrifuged for 35 min at 500 g . Neutrophils were collected from the 60/70% interface, washed and used immediately. Phagocytic targets M. avium TMC 724 was a gift of Dr Chantal Le Chastelier and was grown in Middlebrook 7H9 medium, before labelling with FITC and opsonization [58] . To this end, bacteria (3 × 10 6 ) were washed in PBS before resuspension in 0.3 ml 0.2 M sodium carbonate pH 9.3 containing 0.01% FITC. After 10 min at room temperature (RT), bacteria were washed twice in PBS and then opsonized for 20 min at 37 °C with heat-inactivated AB human serum before two washes with PBS. Tachyzoites of the RH strain of T. gondii expressing GFP [56] were maintained in human foreskin fibroblasts. For phagocytosis assays, extracellular tachyzoites were opsonized by incubation in a 1:10 dilution of heat-inactivated Toxoplasma-seropositive human serum for 30 min at 37 °C. These parasites were washed twice in HBSS before being counted and resuspended in complete Dulbecco’s modified Eagle’s medium (DMEM) for phagocytosis. Zymosan particles were labelled with FITC or rhodamine-isothiocyante (TRITC) using a modification of a published procedure [20] . Zymosan (10 mg) was washed with PBS and resuspended in 0.3 ml 0.2 M sodium carbonate pH 9.3 before adding 1 μl of FITC or TRITC (5 mg ml −1 DMSO (dimethylsulphoxide)) and incubation for 2 h on a rotating wheel at RT. Labelled zymosan was then washed four times with PBS/DMSO (1/1) then four times with PBS. All resuspensions were performed by vortexing and 1 min bath sonication. Latex beads were opsonized with complement as described [20] . In brief, beads were first opsonized with human IgMs (30 μg ml −1 ) for 1 h at 37 °C on a rotating wheel, washed then resuspended in human AB + serum diluted 1/1 with PBS. After 20 min at 37 °C, beads were washed with PBS and used directly. To assay FcγR-mediated phagocytosis, latex beads were opsonized using mouse-IgG (for phagocytosis by RAW 264.7 macrophages) or human-IgG (for phagocytosis by MDMs) [20] . Beads (10 6 μl −1 ) were incubated with 1 mg ml −1 of IgG for 45 min at 37 °C, then washed with PBS and resuspended in PBS/bovine serum albumin (BSA; 1 mg ml −1 ). For SRBCs, 1.10 6 SRBCs μl −1 in opsonization buffer (50% DMEM /50% PBS/BSA 1 mg ml −1 ) received 1 mg ml −1 of rabbit anti-SRBCs. After 45 min at 37 °C, opsonized SRBCs were washed and finally resuspended in opsonization buffer. Phagocytosis assays To assay phagocytosis, monocytes or macrophages were plated on acid-treated coverslips, washed twice with prewarmed DMEM then overlaid with zymosan, opsonized latex beads or SRBCs. Before assaying complement-mediated phagocytosis, MDMs were treated for 15 min with 150 ng ml −1 PMA to activate CR3 (ref. 20 ). RAW 264.7 cells were pretreated with interleukin-4 to increase MR expression [59] 24 h before assaying zymosan phagocytosis. Phagocytic targets were used at a target/macrophage ratio of 10 (SRBCs), 20 ( T. gondii ), 40–50 (beads or M. avium ) or 100 (zymosan). Bacteria and parasites were directly added to cells in complete culture medium. Phagocytosis was synchronized by centrifugation for 1 min at 300 g before incubating the plates at 37 °C for 7–10 min except for complement-mediated phagocytosis (30 min). Plates were then placed on ice and washed before labelling extracellular beads or toxoplasma using fluorescent anti-species antibody for 20 min at 4 °C (ref. 20 ). Extracellular zymosan and M. avium were labelled using specific antibodies. Immunofluorescence using anti-p24 antibodies was performed when using HIV-1-infected cells. Cells were then mounted and imaged using a fluorescent microscope before target counting. Images were randomly acquired. At least 100 cells were examined for each condition and experiments were repeated three times. The mean number of phagocytosed targets was calculated, and results are expressed as percentage of control cells (mean±s.e.m. with n =3 experiments). Line plots (width: five pixels) were generated using Image J. To quantify the number of cells showing GFP–GTPase accumulation at the cup, a line plot was made across the cell and passing through the cup (see Fig. 6a ). Accumulation was considered as significant if fluorescence at the cup was above twofold that observed at the membrane on the opposite side of the cell. At least 20 cups were scored for each condition. To measure the pseudopod length, MDMs were pretreated with 2 nM Tat for 5 h before adding IgG-opsonized beads for 3 min, fixation, permeabilization, staining beads with anti-human fluorescent antibodies and actin with fluorescent phalloidin. Confocal sections were centered on the equatorial plane of the bead. Fifty cups were imaged for each condition and pseudopod length (±s.e.m.) was measured using phalloidin fluorescence and image J. To assay phagocytosis by neutrophils, cells were pretreated with Tat, then washed and resuspended (at 10 6 cells ml −1 ) in Hepes-buffered DMEM containing 30 IgG beads per cell. After 10 min at 37 °C, cells were cooled on ice, centrifuged for 3 min at 300 g , washed with cold PBS and finally centrifuged at 4 °C for 1 min at 250 r.p.m. on alcian blue-coated coverslips. Extracellular beads were then labelled at 4 °C before washes, fixation and mounting. Endocytosis assays Tat or Tat-W11Y (100 nM) was added to human MDMs on ice. After 30 min, cells were washed at 4 °C then incubated at 37 °C for various times. Transferrin-Cy5 (80 nM) was added for the last 40 min. Cells were then washed and processed for detection of Tat and Lamp-1 by immunofluorescence before examination under a confocal microscope. Representative median optical sections were recorded. Co-localization between Tat and Lamp-1 or transferrin was quantified using the Mander’s coefficient calculated using the JACoP plugin of ImageJ. Transactivation assays RAW 264.7 macrophages were transfected in triplicate with 1.5 μg of pGL3-LTR, a vector encoding Firefly luciferase under the control of HIV-1 LTR, 0.25 μg pRL-TK that expresses the Renilla luciferase under the control of the HSV thymidine kinase promoter, with or without 0.25 μg of pcDNA-human cyclin T1. The total DNA for each transfection was normalized to 2 μg with pCI vector (Promega). After 18 h, cells were treated with 100 μM chloroquine and 200 nM Tat or Tat-W11Y. Cells were lysed 24 h later, luciferase activities were measured and transactivation efficiency was calculated as Firefly(Tat)/Renilla(Tat)–Firefly(Ctrol)/Renilla(Ctrol) [19] . Immunofluorescence Cells were washed then fixed in 3.7% paraformaldehyde in PBS before incubation in 50 mM ammonium chloride, and permeabilization with saponin, (0.1% for RAW 264.7 cells and 0.5% for human MDMs). Proteins were revealed by sequential incubation with primary then secondary antibodies (diluted 1:100) for 1 h at RT. To localize PI(4,5)P 2 , a previously optimized procedure was used [60] with minor modifications. Cells were maintained on ice and ice-cold buffers were used throughout the labelling procedure. Following overnight fixation with 4% paraformaldehyde in PBS containing 2 mM EGTA, cells were rinsed with PBS containing 50 mM ammonium chloride, then permeabilized in PBS supplemented with 1 mM MgCl 2 , 1% FBS, 0.1% BSA, 0.2% saponin and 50 mM glycine for 3–4 h. Cells were then labelled with primary antibodies for 4–16 h, rinsed 3 × with permeabilization buffer, labelled for 2 h with secondary antibodies and rinsed before mounting. Cells were viewed under a Leica SPE confocal microscope with a × 63 (NA 1.4) objective. Representative median confocal sections are shown. Image quantification was performed using ImageQuant (GE Healthcare). To quantify PI(4,5)P 2 levels from cell images, the cell perimeter was measured using imageJ and data were normalized to the perimeter of control (EGFP-transfected) cells. Biochemical GTPase activation assay Raw 264.7 macrophages were treated with 10 nM Tat or controls for 5 h. IgG-coated SRBCs were then added to macrophages at a 20:1 ratio. After the indicated time at 37 °C, cells were washed and lysed in 150 mM NaCl, 1 mM Na orthovanadate, 50 mM NaF, 5% glycerol, 1% Triton-X-100, 1 mM dithiothreitol, 50 mM Tris, pH 8.0, supplemented with antiproteases (Complete, Roche). The cell lysate was cleared by centrifugation and an aliquot was saved to quantify total GTPase levels. Purified GST-CRIB-agarose was then added. After three washes in lysis buffer, proteins bound to GST-CRIB were eluted in SDS/polyacrylamide gel electrophoresis sample buffer. Total and activated Cdc42 were then quantified using Western blotting and ImageQuant. Antibodies were diluted 1:3,000 for western blots. Full-size blots are shown in Supplementary Fig. 11 . FRET assay for Cdc42 activation RAW 264.7 macrophages in 35-mm diameter Ibidi glass bottom dishes were transfected with the Cdc42 Raichu probe using Lipofectamine 3000. This probe contains cyan fluorescent protein (CFP), yellow fluorescent protein (YFP), Cdc42 and an activated-Cdc42-binding domain so that intramolecular FRET between CFP and YFP will result of GTPase activation [43] . After 24 h, the medium was replaced by phenol-red free medium containing 1% FBS and IgG-coated SRBCs were added (20 per macrophage). Observation was done using a Nikon TE eclipse inverted microscope of the MRI facilities equipped with a thermal incubation chamber maintained at 37 °C, a mercury lamp, a × 100 (NA 1.49) objective, a cooled digital ImagEM camera and filter wheels for both excitation and emission filters. CFP and FRET 16-bits images were collected every 20 s for 6 min, using CFP excitation filter (426–446 nm) and a YFP emission filter for the FRET image as detailed [43] . Preliminary experiments were performed to find illumination conditions where bleaching of CFP and YFP was <10% of the signal intensity over the timescale of the experiment. The microscope was piloted using Metamorph (Universal Imaging) and FRET efficiency calculation was performed as described [43] using an ImageJ plugin written by Virginie Georget (MRI facility). In brief, the background was subtracted from both the CFP and FRET images, before applying a threshold and creating the FRET/CFP ratio image. Pseudocolors (Lookup Table-Fire in ImageJ) were used to show the different ratio values on the images. White corresponds to the highest FRET intensity. Scanning electron microscopy MDMs on coverslips were fixed with 2.5% glutaraldehyde in 0.1 M phosphate buffer, pH 7.2 before washing, dehydration using EtOH and treatment with hexamethyldisilazane. Samples were viewed under an Hitachi S4000 microscope using a 45° tilt angle. How to cite this article: Debaisieux, S. et al . HIV-1 Tat inhibits phagocytosis by preventing the recruitment of Cdc42 to the phagocytic cup. Nat. Commun. 6:6211 doi: 10.1038/ncomms7211 (2015).